Collective fluorescence switching of counterion-assembled dyes in polymer nanoparticles The current challenge in the field of fluorescent nanoparticles (NPs) for bioimaging is to achieve extreme brightness and external control of their emission using biodegradable materials. Here we propose a new concept of fluorescent polymer NPs, doped with ionic liquid-like salts of a cationic dye (octadecyl rhodamine B) with a bulky hydrophobic counterion (fluorinated tetraphenylborate) that serves as spacer minimizing dye aggregation and self-quenching. The obtained 40-nm poly( D , L -lactide- co -glycolide) NPs containing up to 500 dyes are brighter than quantum dots and exhibit photo-induced reversible on/off fluorescence switching, never reported for dye-doped NPs. We show that this collective switching of hundreds of dyes is due to ultrafast excitation energy transfer and can be used for super-resolution imaging. These NPs, being spontaneously endocytosed by living cells, feature high signal-to-noise ratio and absence of toxicity. The counterion-based concept opens the way to a new class of nanomaterials for sensing, imaging and light harvesting. Fluorescent nanoparticles (NPs) constitute the most promising platforms for the design of ultrabright multifunctional devices for imaging, diagnostics and therapy [1] . This field is currently dominated by inorganic NPs, such as quantum dots [2] , [3] , dye-doped silica [4] and carbon dots [5] , which show very bright fluorescence but suffer from lack of biodegradability and poor flexibility for encapsulation of molecules, limiting their biomedical applications. Organic dye-doped NPs are excellent candidates to overcome these limitations. Notably, NPs based on biodegradable polymers, such as poly( D,L -lactide- co -glycolide) (PLGA), are known for many years as drug carriers [6] , but the first examples of highly fluorescent dye-doped PLGA NPs appeared only recently [7] , [8] . The main challenge in the design of dye-doped NPs is confining the dyes inside a particle at extremely high concentrations without self-quenching. Indeed, being flat aromatic structures, dyes tend to π -stack into poorly fluorescent aggregates (H-aggregates) [9] . Recent reports showed remarkable exceptions [10] , suggesting that the key to design highly fluorescent NPs is to engineer dye assemblies with proper inter-fluorophore distance and orientation. The other fundamental phenomenon observed at high dye concentrations is excitation energy transfer (EET) (also called exciton diffusion) [11] . EET shuttles the energy in multi-chromophoric systems for photosynthesis [12] , artificial-light harvesting [13] and photovoltaics [14] . Ultrafast EET ensures collective behaviour of multiple fluorophores, allowing their simultaneous quenching, so-called superquenching, reported so far only for conjugated polymers [15] , [16] and J-aggregates [17] , and used for signal amplification in chemo and biosensors [15] , [16] . Collective behaviour is especially exemplified by on/off switching (also called blinking), a process normally observed for single emitters such as individual fluorophores [18] and quantum dots [19] . The phenomenon of blinking in conjugated polymers [20] , dendrimers [21] , photosynthetic centres [12] and J-aggregates [22] shows that due to ultrafast EET, up to 100 fluorophores could be collectively turned off by a single energy trap [20] , [22] . However, collective switching has never been reported for dye-doped NPs. To achieve collective on/off behaviour inside NPs, dyes should undergo very fast EET with minimized self-quenching. To prevent formation of non-fluorescent aggregates, fluorophores are usually modified by bulky side chains [23] , [24] . However, these side chains, being attached ‘in-plane’ of the flat fluorophore, cannot completely abolish its π -stacking. An original alternative is to use ionic dyes in the form of salts with hydrophobic bulky counterions, thus changing the dye topology from planar to three-dimensional. In pure form, such salts were described as ‘frozen ionic liquids’ with appreciable fluorescence, which confirms that the counterion can prevent π -stacking of the dyes [25] , [26] . The tetraphenyl borate (TPB) anion and its fluorinated analogues, used as ionophores in polymeric cation-sensitive electrodes [27] , [28] , are particularly interesting counterions due to their bulky tetrahedral structure. However, so far, no attempts were made to use TPBs for encapsulation of cationic dyes into polymer NPs. In the present work, we show that TPB and especially its fluorinated analogues can strongly decrease the aggregation and self-quenching of a classical cationic dye (rhodamine B derivative) in different polymer matrices. In the case of PLGA, 40-nm NPs encapsulating up to 500 dyes are obtained, which are several times brighter than quantum dots. Remarkably, these NPs show nearly complete and reversible on/off fluorescence switching, a phenomenon that has never been reported for dye-doped NPs. Fluorescence anisotropy studies suggest that this collective behaviour of large dye ensembles is due to ultrafast EET propagating through the whole particle. Owing to this unique switching property, it becomes possible to use dye-doped NPs for super-resolution imaging by direct stochastic optical reconstruction microscopy (dSTORM). Furthermore, cellular studies show that these NPs, being internalized by endocytosis, are not toxic and feature high signal-to-noise ratio in fluorescence microscopy. Preparation of dye salts and NPs Three hydrophobic bulky anions were selected as counterions for apolar cationic octadecyl rhodamine B (R18, Fig. 1 ), namely the parent TPB and two analogues, bearing one (F1-TPB) or five (F5-TPB) fluorines per phenyl ring. The salts 1 , 2 and 3 of the R18 dye with these counterions were obtained from the perchlorate salt using ion exchange, followed by purification. According to thin layer chromatography ( Supplementary Fig. 1 ), the TPB salts are much more hydrophobic (higher Rf mobility) than R18 perchlorate, with R18/F5-TPB being the most hydrophobic. 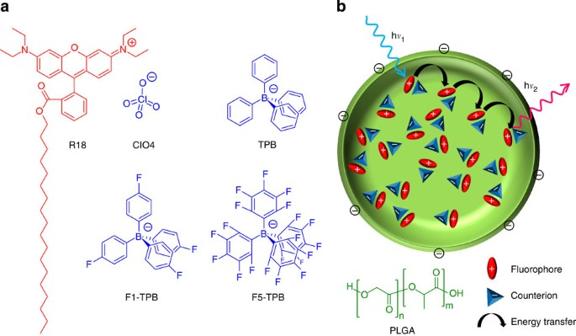Figure 1: Design of dye-doped fluorescent NPs using bulky counterions. (a) Chemical structures of rhodamine B octadecyl ester (R18) and its different counterions: perchlorate (ClO4), tetraphenylborate (TPB), tetrakis(4-fluorophenyl)borate (F1-TPB) and tetrakis(pentafluorophenyl)borate (F5-TPB). (b) Schematic representation of PLGA NPs loaded with these dye salts. Figure 1: Design of dye-doped fluorescent NPs using bulky counterions. ( a ) Chemical structures of rhodamine B octadecyl ester (R18) and its different counterions: perchlorate (ClO4), tetraphenylborate (TPB), tetrakis(4-fluorophenyl)borate (F1-TPB) and tetrakis(pentafluorophenyl)borate (F5-TPB). ( b ) Schematic representation of PLGA NPs loaded with these dye salts. Full size image PLGA NPs obtained by nano-precipitation [29] , [30] of PLGA from acetonitrile solution in aqueous buffer were 37 (±3) nm in diameter with a narrow size distribution (PdI≤0.12), according to dynamic light scattering (DLS) data ( Fig. 2a ), and negative surface charge (−60 mV, Supplementary Table 1 ). To obtain dye-doped NPs, R18 with a given counterion was added to the PLGA solution in acetonitrile (0.1 to 5 wt% with respect to PLGA) and the same nano-precipitation protocol was used. For the parent R18 perchlorate, a rapid increase of the particle size was observed on increase in the dye content ( Fig. 2a ). Remarkably, the TPB-type counterions minimized the undesired influence of dye loading on the particle size, while for F5-TPB this influence was already absent. We speculate that R18 perchlorate, being amphiphilic, can accumulate at the water–PLGA interface of NPs. In contrast, R18 salts with hydrophobic TPB and especially its fluorinated analogues are highly apolar, which allows their encapsulation without modifying their negatively charged surface as confirmed by zeta potential data ( Supplementary Table 1 ). 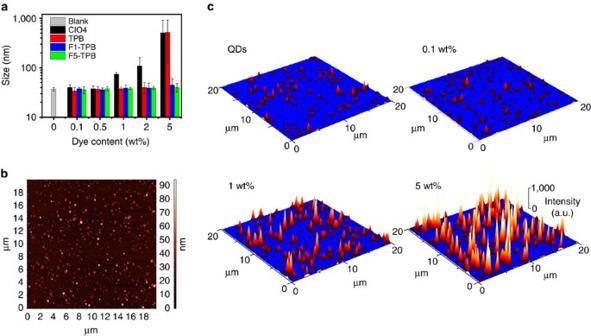Figure 2: Size and fluorescence brightness of dye-doped NPs. (a) Size of PLGA NPs versus dye content for R18 with different counterions as measured by DLS. The experiment was replicated four times. (b) AFM image of NPs loaded with 1 wt% R18/F5-TPB deposited on a polyethyleneimine layer. (c) Fluorescence microscopy images of quantum dots (QDs, QDot 605 streptavidin conjugate) and NPs containing 0.1, 1, and 5 wt% of R18/F5-TPB. The brightness of single QDs and NPs at 0.1, 1 and 5 wt% dye loading was 23 (±7), 10 (±1.5), 70 (±7) and 140 (±9), respectively. Micrographs were obtained under the same conditions of illumination and recording; at least 200 particles were analysed per condition; the errors correspond to s.e.m. Figure 2: Size and fluorescence brightness of dye-doped NPs. ( a ) Size of PLGA NPs versus dye content for R18 with different counterions as measured by DLS. The experiment was replicated four times. ( b ) AFM image of NPs loaded with 1 wt% R18/F5-TPB deposited on a polyethyleneimine layer. ( c ) Fluorescence microscopy images of quantum dots (QDs, QDot 605 streptavidin conjugate) and NPs containing 0.1, 1, and 5 wt% of R18/F5-TPB. The brightness of single QDs and NPs at 0.1, 1 and 5 wt% dye loading was 23 (±7), 10 (±1.5), 70 (±7) and 140 (±9), respectively. Micrographs were obtained under the same conditions of illumination and recording; at least 200 particles were analysed per condition; the errors correspond to s.e.m. Full size image Atomic force microscopy (AFM) analysis of dye-doped NPs immobilized on a glass surface ( Fig. 2b ) yielded a particle size of 37 (±5) nm, in good agreement with the DLS data. Combined AFM/fluorescence microscopy ( Supplementary Fig. 2 ) revealed that the particles and the fluorescence were co-localized, confirming the fluorophore encapsulation inside the NPs. Photophysics of NPs in solution Irrespective of their counterion, the dye salts alone showed a very weak fluorescence in buffer with fluorescence quantum yields (QYs)<2%, which is probably related to their aggregation induced self-quenching in water [31] . After encapsulation into NPs, the situation was quite different ( Fig. 3 and Supplementary Fig. 3 ). At low dye loading (<1 wt%), all four dye salts showed very high QY, comparable or better than that in methanol. At higher loading, QY dropped rapidly for R18 perchlorate and, to a lesser extent, for TPB and F1-TPB counterions, leading to less fluorescent NPs. The only exception was the R18 salt with the perfluorinated F5-TPB, which preserved relatively high QY and, thus, led to a continuous increase in NP brightness up to 5 wt% loading ( Fig. 3a ). Remarkably, encapsulation of the R18/F5-TPB salt into NPs composed of other polymers, such as polycaprolactone, poly(methyl methacrylate) and polystyrene, also gave very efficient fluorescence at high dye loading ( Supplementary Fig. 4 ). The F5-TPB anion is thus able to reduce self-quenching of the cationic dye in a variety of polymer matrices. To verify whether the unique behaviour of the F5-TPB counterion stems from the fluorination alone, we encapsulated R18 perchlorate together with 1–4 mole eq. of hexafluorobenzene, an analogue of the aromatic residues in F5-TPB. However, the presence of hexafluorobenzene did not influence the self-quenching of R18 perchlorate ( Supplementary Fig. 5 ), indicating that ionic interactions of the bulky fluorinated counterion are essential for preventing dye aggregation. Remarkably, fluorescence microscopy of PLGA NPs immobilized on a glass surface ( Fig. 2c ) further revealed that our NPs loaded with 1 and 5 wt% R18/F5-TPB were, respectively, three- and sixfold brighter than quantum dots under identical conditions ( Fig. 2c ). 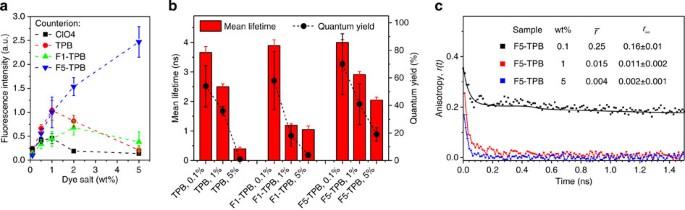Figure 3: Fluorescence properties of dye-doped NPs for different counterions. (a) Fluorescence intensities (λex=530 nm) versus dye salt concentration inside NPs. (b) Mean fluorescence lifetimes and QYs of these systems. The experiments were replicated at least three times. The error bars correspond to s.e.m. (c) Time-resolved anisotropy decays of various dye-doped NPs. The steady-state anisotropyand residual anisotropy (r∞) are given in the inset. For 0.1 wt% R18/F5-TPB, the corresponding fit is given, and the residual anisotropy corresponds to the fitted value. For 1 and 5 wt% R18/F5-TPB, the lines are guides to the eye. In these cases the residual anisotropies were determined as mean value of the anisotropy between 1 and 4 ns, and the given error is the s.e.m. Figure 3: Fluorescence properties of dye-doped NPs for different counterions. ( a ) Fluorescence intensities ( λ ex =530 nm) versus dye salt concentration inside NPs. ( b ) Mean fluorescence lifetimes and QYs of these systems. The experiments were replicated at least three times. The error bars correspond to s.e.m. ( c ) Time-resolved anisotropy decays of various dye-doped NPs. The steady-state anisotropy and residual anisotropy ( r ∞ ) are given in the inset. For 0.1 wt% R18/F5-TPB, the corresponding fit is given, and the residual anisotropy corresponds to the fitted value. For 1 and 5 wt% R18/F5-TPB, the lines are guides to the eye. In these cases the residual anisotropies were determined as mean value of the anisotropy between 1 and 4 ns, and the given error is the s.e.m. Full size image At temperatures well below the glass transition of the PLGA matrix [32] , the dye molecules are thought to be immobilized, so that the decrease of QY at higher dye loading is probably related to formation of non-fluorescent aggregates [31] . Their presence in PLGA NPs is supported by the observed changes in the absorption spectra ( Supplementary Figs 6 and 7 ), namely (1) band broadening, (2) increased contribution of the short-wavelength shoulder around 530 nm [31] and (3) red shift of the absorption maximum [33] , [34] , although these changes were less pronounced than for pure salts in water ( Supplementary Fig. 8 ). Remarkably, only for R18/F5-TPB in PLGA NPs, the absorption and the fluorescence maxima were close to those in methanol ( Supplementary Figs 6–11 ), indicating the lowest dye aggregation and explaining the highest observed QY values. To further understand the mechanism of self-quenching, we performed fluorescence lifetime measurements ( Fig. 3b , Supplementary Fig. 12 and Supplementary Table 2 ). At 0.1 wt% of dye with all three TPBs, we observed a nearly single-exponential decay, with a lifetime value about twice that of R18 perchlorate in methanol, in line with the difference in QY and the expected confinement of R18 in the rigid PLGA matrix. On increasing the dye loading, the mean lifetimes decreased ( Fig. 3b ) in the order TPB>F1-TPB>F5-TPB, in good agreement with the corresponding losses in QY, due to the appearance of short-lived decay components from poorly fluorescent dye aggregates. Importantly, for F5-TPB the contribution of the long-lived decay time to the emission remained dominant even at 5 wt% loading (74%, Supplementary Fig. 13 ), confirming minimized self-quenching with this counterion. Having fluorescent NPs at relatively high dye loading, we further studied their EET. As EET between randomly oriented fluorophores results in light depolarization [34] , [35] , we performed fluorescence steady-state and time-resolved anisotropy measurements ( Fig. 3c ). At 0.1 wt% of R18 with all three TPB-type counterions, NPs showed high steady-state anisotropy values, ~0.25, indicating that the fluorophores are well immobilized inside NPs ( Supplementary Table 3 ). At ≥1 wt% dye content, the steady-state anisotropy values decreased strongly and this effect was particularly drastic for F5-TPB, where it dropped >60-fold ( Fig. 3c ). Time-resolved anisotropy decay data further suggested extremely fast EET-driven light depolarization on the timescale <60 and <20 ps for 1 and 5 wt% of R18/F5-TPB, respectively ( Fig. 3c ). Remarkably, the residual anisotropy values ( r ∞ ) for these NPs were extremely low, in good agreement with the steady-state anisotropy ( Fig. 3c ). The r ∞ values are inversely proportional to the number of fluorophores involved in EET ( N = r 0 / r ∞ ) [36] , [37] , where r 0 is the fundamental anisotropy (0.37 for rhodamine B). Therefore, we can roughly estimate that for 1 and 5 wt% loading with R18/F5-TPB, around 40 and 200 fluorophores, respectively, were engaged in EET. Together with the ultrafast anisotropy decay, this suggested that the excitation energy can readily delocalize over the whole particle, which means over ~100 and 500 dyes for 1 and 5 wt% loading, respectively. This was clearly not the case at lower R18/F5-TPB loading and for the other counterions, where the residual anisotropy was much larger and/or the anisotropy decay was much slower ( Supplementary Fig. 14 ). It should be noted that possible heterogeneity of encapsulation sites in PLGA NPs cannot explain this drastic loss of anisotropy. Indeed, R18/F-TPB, a close analogue of R18/F5-TPB, which should occupy similar polymer sites, did not show this anisotropy loss ( Supplementary Table 3 ). Moreover, at high dye loading the anisotropy decay for R18/F5-TPB is much faster compared with even freely rotating tetramethylrhodamine in water (180 ps). Single-particle measurements As this ultrafast delocalization of the excitation energy was expected to lead to a collective behaviour of the dyes at the level of the whole NP, we monitored the time-dependent emission of individual NPs immobilized on glass surfaces by single molecule fluorescence microscopy. For NPs loaded with 1 and 5 wt% of R18 with the F5-TPB counterion, we observed reversible on/off fluorescence switching (blinking) of the NPs ( Supplementary Movie 1 ), a phenomenon that has never been reported to date for dye-doped NPs. Typical transients for individual NPs containing 0.1 to 5 wt% of F5-TPB are shown in Fig. 4a . At the lowest dye loading (0.1 wt%), no on/off-switching was observed, but only small variations of the fluorescence intensity. At 1 and 5 wt%, on/off-switching was observed for >90% of the NPs. During the off-periods, their fluorescence intensity fell close to the background level, indicating that nearly all of the encapsulated fluorophores (100 and 500, respectively) turned off simultaneously. Moreover, during the measurement time, nearly all NPs after a turn off went back to the on-state at least once ( Supplementary Fig. 15 ). To further determine the number of fluorophores involved in the collective on/off switching, we measured the absolute number of fluorophores emitting in the on-state [22] by comparing the brightness of immobilized NPs to that of standard fluorescent polystyrene beads with known brightness. Taking into account the QY of our NPs with 1 and 5 wt% R18/F5-TPB loading, the average number of emitting fluorophores per particle was 105 (±20) and 500 (±50), respectively. This means that both types of NPs showed an exceptional collective behaviour with practically all of their fluorophores switching simultaneously. 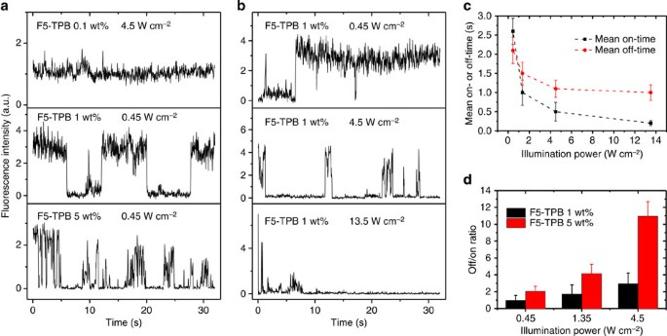Figure 4: Fluorescence on/off switching of dye-doped NPs. (a,b) Emission transients of NPs, with 32-ms time resolution. Dependence of emission transients on R18/F5-TPB concentration (a) and illumination power (b). (c) Dependence of the mean on- and off-state duration on the illumination power for NPs loaded with 1 wt% R18/F5-TPB. Dashes are guides to the eye. (d) The mean off-to-on ratio of PLGA NPs for different R18/F5-TPB dye loadings and illumination powers. At least 200 particles per condition were analysed for the emission transients. The error bars correspond to s.e.m. Figure 4: Fluorescence on/off switching of dye-doped NPs. ( a , b ) Emission transients of NPs, with 32-ms time resolution. Dependence of emission transients on R18/F5-TPB concentration ( a ) and illumination power ( b ). ( c ) Dependence of the mean on- and off-state duration on the illumination power for NPs loaded with 1 wt% R18/F5-TPB. Dashes are guides to the eye. ( d ) The mean off-to-on ratio of PLGA NPs for different R18/F5-TPB dye loadings and illumination powers. At least 200 particles per condition were analysed for the emission transients. The error bars correspond to s.e.m. Full size image Comparison of transients recorded with NPs in various conditions ( Fig. 4a,b ) revealed that the frequency of the switching process was higher for the 5 wt% F5-TPB NPs than for the 1 wt% NPs and that their blinking depended on the illumination power ( Fig. 4b ). An analysis of 200 NPs showed that with increase in laser power, the mean duration of the on-state (and to some extent of the off-state) decreased ( Fig. 4c ), while the contribution of the off-state (off/on ratio) increased ( Fig. 4d ), suggesting that the switching of NPs is controlled by illumination. Therefore, the observed switching is a result of photo-induced processes, for example, electron transfer and intersystem crossing, as reported for single fluorophores and quantum dots [38] , [39] . Furthermore, similarly to these classical blinking systems [40] , [41] , the frequency of the on- and off-times followed a power law behaviour ( Supplementary Fig. 16 ). A remarkable feature of our R18/F5-TPB NPs is that the off/on ratio can be significantly increased at higher dye loading ( Fig. 4d ), which is important for their potential application in super-resolution imaging (see below). For TPB and F1-TPB at 1 wt% loading, the typical transients showed no blinking ( Supplementary Fig. 17 ), but only small and slow variations of the fluorescence intensity. Super-resolution imaging On/off switching of NPs is of particular interest for super-resolution imaging, such as dSTORM [42] , [43] . As dSTORM requires emitters that feature much longer off-state compared with the on-state [44] , [45] , we have chosen our 5 wt% R18/F5-TPB NPs, which meets this requirement best ( Fig. 4d ). Application of a super-localization procedure to our NPs immobilized on glass surfaces gave images where the point-spread functions of single NPs had a width at half-maximum of 35±7 nm ( Fig. 5 ), which correlates well with AFM and DLS data. Blinking of our NPs allowed us to detect single NPs and resolve them at interparticle distances below the diffraction limit ( Fig. 5d,e ). This is the first proof-of-principle demonstration of dSTORM imaging of dye-doped NPs exploiting collective blinking of hundreds of dyes, which should improve the sensitivity of the method. Indeed, our super-resolution images were acquired at much lower laser power (4.5 W cm −2 ) than those typically used for single dyes. 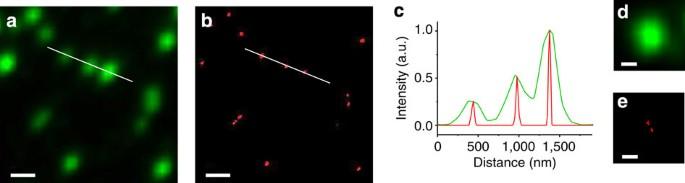Figure 5: Super-resolution imaging using PLGA NPs loaded with 5 wt% R18/F5-TPB NPs. (a) Standard TIRF image of immobilized NPs, (b) the same field after applying a super-localization procedure (scale bar, 500 nm), (c) intensity profiles along the line marked in (a) green and (b) red, showing the reduction in the width of the point spread function (PSF). Standard TIRF image (d) and the same field after using a super-localization procedure (e) showing the resolving power. Scale bar, 200 nm. Figure 5: Super-resolution imaging using PLGA NPs loaded with 5 wt% R18/F5-TPB NPs. ( a ) Standard TIRF image of immobilized NPs, ( b ) the same field after applying a super-localization procedure (scale bar, 500 nm), ( c ) intensity profiles along the line marked in ( a ) green and ( b ) red, showing the reduction in the width of the point spread function (PSF). Standard TIRF image ( d ) and the same field after using a super-localization procedure ( e ) showing the resolving power. Scale bar, 200 nm. Full size image Interaction with living cells and cytotoxicity Finally, to explore the applicability of our new particles to cellular imaging applications, we incubated the 1 wt% R18/F5-TPB NPs with living cells and imaged them by confocal microscopy ( Fig. 6 ). Already after 3 h of incubation, the NPs can be observed inside the cells as very bright multiple spots ( Fig. 6a ). These spots co-localized well with LysoTracker Green DND-26 ( Fig. 6b and Supplementary Fig. 18 ), indicating that the particles entered into the cells by endocytosis. This conclusion was confirmed by measurements at 4 °C, which showed no signs of NPs internalization ( Supplementary Fig. 19 ). Remarkably, despite the use of very low particle concentration (~0.15 nM, that is ~15 nM of R18) the signal obtained from the endosomes was >50-fold stronger than in the rest of the cytoplasm, while for 50 nM LysoTracker the signal-to-background ratio was much lower (~5-fold). This excellent contrast is clearly due to the high brightness of our NPs, also suggesting that the encapsulated dyes do not undergo a detectable leaching from NPs into the cytoplasm (even after 1 week of incubation, Supplementary Fig. 20 ). Moreover, PLGA NPs without and with 1 and 5 wt% of the loaded dye showed no signs of cytotoxicity even at the highest concentrations tested, which are >100-fold larger than used for imaging ( Fig. 6c and Supplementary Fig. 21 ). 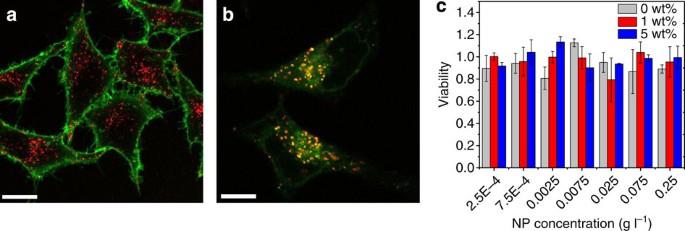Figure 6: Imaging and toxicity of dye-doped NPs in HeLa cells. (a) Micrograph of HeLa cells cultured for 3 h in the presence of 1 wt% R18/F5-TPB NPs and for 10 min in the presence of wheat-germ agglutinin-Alexa488 for labelling of cell membranes. Scale bar, 20 μm. (b) Micrograph of HeLa cells cultured for 3 h with 1 wt% R18/F5-TPB NPs and for 30 min with LysoTracker Green DND-26. Scale bar, 10 μm. The micrographs inaandbwere obtained using a confocal microscope with excitation at 532 nm (red) and 488 nm (green) to image NPs and WGA-Alexa488 (a) or LysoTracker (b), respectively. (c) Viability of HeLa cells exposed for 24 h to different concentrations of PLGA NPs loaded with 0, 1 and 5 wt% R18/F5-TPB. The highest concentration of the 5 wt% NPs corresponds to a 10-μM concentration of the dye, that is >500-fold larger than the highest concentration used for cellular imaging. Cell viability was tested in triplicate using MTT. The error bars correspond to s.e.m. Figure 6: Imaging and toxicity of dye-doped NPs in HeLa cells. ( a ) Micrograph of HeLa cells cultured for 3 h in the presence of 1 wt% R18/F5-TPB NPs and for 10 min in the presence of wheat-germ agglutinin-Alexa488 for labelling of cell membranes. Scale bar, 20 μm. ( b ) Micrograph of HeLa cells cultured for 3 h with 1 wt% R18/F5-TPB NPs and for 30 min with LysoTracker Green DND-26. Scale bar, 10 μm. The micrographs in a and b were obtained using a confocal microscope with excitation at 532 nm (red) and 488 nm (green) to image NPs and WGA-Alexa488 ( a ) or LysoTracker ( b ), respectively. ( c ) Viability of HeLa cells exposed for 24 h to different concentrations of PLGA NPs loaded with 0, 1 and 5 wt% R18/F5-TPB. The highest concentration of the 5 wt% NPs corresponds to a 10-μM concentration of the dye, that is >500-fold larger than the highest concentration used for cellular imaging. Cell viability was tested in triplicate using MTT. The error bars correspond to s.e.m. Full size image We showed that bulky fluorinated organic counterions can drastically reduce π -stacking (aggregation) and hence self-quenching of a classical cationic dye in polymer NPs. This counterion-based concept allows for preparation of dye-doped PLGA NPs of <40-nm size that are three- to sixfold brighter than quantum dots. Moreover, it works also in other polymer matrices, such as polycaprolactone, poly(methyl methacrylate) and polystyrene, and we expect that it can be also extended in principle to other ionic dyes. Therefore, this concept can be considered as a generic solution to the fundamental problem of dye aggregation and self-quenching [9] , [46] , [47] . It should be added that the counterion also enables dye encapsulation without modification of the particle surface, which is required for preparation of small and stable NPs. The second important finding is the collective behaviour of several hundred fluorescent dyes inside NPs resulting in on/off fluorescence switching (blinking) of the particles. The observed on/off switching behaviour correlates well with our fluorescence anisotropy data. Indeed, only for F5-TPB at 1–5 wt% loading, NPs exhibited both on/off switching and very fast anisotropy decay with low residual anisotropies. The blinking hence occurred only in NPs, where the excitation energy was rapidly delocalized. Next, a single dark state, which for rhodamine dyes is probably of radical nature [48] , could quench the whole particle. The observed EET process in 1 wt% F5-TPB NPs with a time constant of <60 ps is surprisingly fast compared with other dye-doped systems. Thus, for Lumogen Red at similar dye loading in a poly(methyl methacrylate) matrix, the anisotropy decay time was ~40-fold slower [34] . For Lumogen Red, the anisotropy decay time was well described by a homo-Förster resonance energy transfer mechanism of EET, assuming an isotropic distribution of the dye inside the polymer [34] : where τ a is the anisotropy decay time, τ 0 is the fluorescence lifetime of the fluorophore in the absence of EET, R 0 is the Förster distance of homo-Förster resonance energy transfer and C is the concentration of the fluorophore (molecules per nm 3 ). However, using the calculated R 0 for R18 (5.2 nm), equation (1) predicts an anisotropy decay time of 500 ps for our 1 wt% R18/F5-TPB NPs, which is about tenfold longer than what was experimentally observed. This implies that the real inter-fluorophore distance inside the polymer is smaller than the average value l iso expected from the isotropic distribution of the dyes ( , l iso =3.4 nm for 1 wt% loading) [34] . We hence speculate that inside NPs the R18 molecules are assembled into domains by the F5-TPB counterions that ‘bridge’ the cationic dyes together in the close proximity needed for ultrafast EET ( Fig. 7 ), while preventing them from π -stacking into non-fluorescent aggregates. The chemical structure of R18/F5-TPB, with its bulky hydrophobic ions, is typical for (frozen) ionic liquids [25] , which suggests that it can undergo an electrostatically driven short-range ordering inside the PLGA matrix ( Fig. 7 ). Among the studied counterions, F5-TPB, being the bulkiest, the most hydrophobic and having the highest negative charge density at its surface due to its highly electronegative fluorines, is thought to be the best counterion to favour this ordering. Complete on/off switching can only be observed in systems that behave similar to a single exciton, namely single dye molecules [18] , quantum dots [19] , [40] , dye dendrimers [21] , [49] , J-aggregates [22] or single chains of conjugated polymers [20] . Here we obtained the first dye-doped NPs undergoing complete on/off switching due to collective dye behaviour, which can be realized even for ensembles of 500 dyes. This exceptional collectiveness of dyes, where a single energy acceptor harvests efficiently the energy from a large ensemble of donors, can lead to new on/off switching devices for sensing [15] , [16] , [50] and nanomaterials for light harvesting [47] , [51] , [52] . 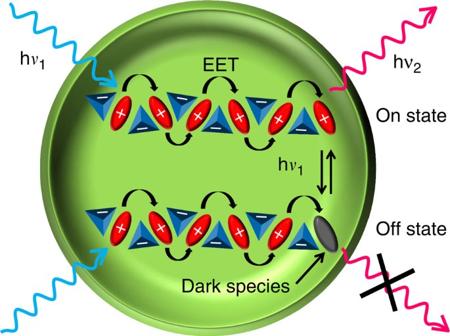Figure 7: Proposed model of the counterion-assembled dyes inside NPs. Short-range ordering (shown as one-dimensional for simplicity) of R18 cations (red) by the F5-TPB counterion (blue) inside the polymer matrix (green) prevents dye aggregation and leads to the short inter-fluorophore distance suggested by the ultrafast EET. Dark species (grey) generated by light turn off the whole ensemble of dyes coupled by EET leading to on/off switching. Figure 7: Proposed model of the counterion-assembled dyes inside NPs. Short-range ordering (shown as one-dimensional for simplicity) of R18 cations (red) by the F5-TPB counterion (blue) inside the polymer matrix (green) prevents dye aggregation and leads to the short inter-fluorophore distance suggested by the ultrafast EET. Dark species (grey) generated by light turn off the whole ensemble of dyes coupled by EET leading to on/off switching. Full size image The observed switching phenomenon allowed imaging of our NPs with sub-diffraction resolution using a dSTORM technique [42] , [43] . As the switching process involves >100 dyes simultaneously, we expect that the sensitivity of dSTORM could be improved many-fold by using our NPs. Although the size of these NPs (40 nm) is much larger than that of single dye molecules, it remains close to the typical resolution of dSTORM with organic dyes (~20 nm) [43] . Moreover, we foresee that a decrease in the particle size to 15–20 nm is a feasible task. Finally, we also showed that these particles could be applied for cellular imaging, featuring high signal-to-noise ratio, minimal dye leaching and absence of toxicity. Compared with the best reported biodegradable dye-doped NPs [7] , [8] , our NPs are smaller (35 nm versus 60 nm) and the QY of the encapsulated dyes is much higher (20% for 5 wt% dye loading in our NPs versus only 2% for 3 wt% loading in the reference dye-doped NPs [8] ). However, the most important feature is the collective on/off behaviour of dyes in our NPs, which has not been reported for any dye-doped NPs, opening new possibilities for super-resolution imaging and biosensing. The finding of unique properties together with the importance of PLGA NPs in biomedical research [53] make our particles an attractive biodegradable alternative to quantum dots. Materials PLGA (lactide 50 mole%, glycolide 50 mole%, M n 24,000; PDI 1.7), rhodamine B octadecyl ester perchlorate (≥98.0%), sodium tetraphenylborate (≥99.5%), sodium tetrakis(4-fluorophenyl)borate dihydrate (≥97.0%), lithium tetrakis(pentafluorophenyl)borate ethyl etherate, acetonitrile (≥99.5%) were purchased from Sigma-Aldrich and used as received. Sodium phosphate monobasic (>99.0%, Sigma-Aldrich) and sodium phosphate dibasic dihydrate (>99.0%, Sigma-Aldrich) were used to prepare 20 mM phosphate buffer solutions at pH 7.4. MilliQ-water (Millipore) was used in all experiments. Synthesis of dye salts The salts of octadecyl rhodamine B with different counterions were obtained by ion exchange followed by purification. NMR spectra were recorded at 20 °C on Bruker Avance III 400 or 500 MHz spectrometer. Mass spectra were obtained using an Agilent Q-TOF 6520 mass spectrometer. Rhodamine B octadecyl ester tetraphenylborate 1 To 98 mg of sodium tetraphenylborate (286 μmol, 50 eq.) dissolved in 4 ml of acetonitrile were added rapidly 4.5 mg of rhodamine B octadecyl ester perchlorate (5.7 μmol). After evaporation of the solvent, the raw product was purified by thin layer chromatography (eluent: dichloromethane/methanol: 95/5). After re-dissolution, filtration and drying under vacuum, the product was obtained as a purple solid (4 mg, yield 70%). 1 H NMR (400 MHz, DMSO-d6): δ 8.23 (dd, J =7.8 Hz, J =1.2 Hz, 1H), 7.86 ( m , 2H), 7.80–6.60 ( m , 27H), 3.88 ( t , J =6.1 Hz, 2H), 3.63 ( q , J =7.2 Hz, 8H), 1.35–0.80 ( m , 47H); 13 C NMR (100 MHz, DMSO-d6): δ 164.5, 162.8 ( q , J =49 Hz), 157.1, 156.6, 154.6, 135.5, 132.5, 132.1, 130.4, 130.3, 129.9, 129.8, 129.3, 124.7, 120.9, 114.0, 112.4, 95.3, 64.6, 44.8, 30.7, 28.5, 28.4, 28.2, 28.1, 28.0, 27.2, 24.7, 21.5, 13.4, 11.9; 11 B NMR (128 MHz, DMSO-d6): δ −6.67; HRMS ( m/z ): [M] + calcd. for C 46 H 67 N 2 O 3 , 695.5146; found, 695.5156; [M] − calcd. for C 24 H 20 B, 319.1664; found, 319.1666. Rhodamine B octadecyl ester tetrakis(4-fluorophenyl)borate 2 To 31 mg of sodium tetrakis(4-fluorophenyl)borate dihydrate (69 μmol, 20 eq.) dissolved in 2 ml of acetonitrile were added rapidly 2.8 mg of rhodamine B octadecyl ester perchlorate (3.5 μmol) in 0.6 ml acetonitrile. After evaporation of the solvent, the raw product was purified by thin layer chromatography (eluent: dichloromethane/methanol: 95/5). After re-dissolution, filtration and drying under vacuum, the product was obtained as a purple solid (2.5 mg, yield 66%). 1 H NMR (400 MHz, CD 3 OD): δ 8.33 (dd, J =7.5 Hz, J =1.4 Hz, 1H), 7.85 ( m , 2H), 7.45 (dd, J =7.5 Hz, J =1.3 Hz, 1H), 7.20–7.10 ( m , 10H), 7.07 (dd, J =9.5 Hz, J =2.3 Hz, 2H), 7.01 ( d , J =2.3 Hz, 2H), 6.66 ( m , 8H), 3.96 ( t , J =6.3 Hz, 2H), 3.68 ( q , J =7.0 Hz, 8H), 1.33 ( t , J =7.0 Hz, 12H), 1.30–0.85 ( m , 35H); 13 C NMR (125 MHz, CD 3 OD): δ 166.9, 161.3 ( d , J =236 Hz), 160.1, 159.6 ( q , J =49 Hz), 159.3, 157.1, 137.9, 134.5, 134.0, 132.4, 132.3, 131.9, 131.6, 131.5, 115.5, 114.8, 112.6 ( d , J =18 Hz), 97.2, 66.8, 46.8, 33.1, 30.8, 30.7, 30.5, 30.4, 30.3, 29.4, 26.9, 23.7, 14.5, 12.8; 11 B NMR (128 MHz, CD 3 OD): δ −7.65 ( m ); 19 F NMR (160 MHz, CD 3 OD): δ −126 ( s ); HRMS ( m/z ): [M] + calcd. for C 46 H 67 N 2 O 3 , 695.5146; found, 695.5151; [M] − calcd. for C 24 H 16 BF 4 , 391.1287; found, 391.1278. Rhodamine B octadecyl ester tetrakis(pentafluorophenyl)borate 3 To 21 mg of lithium tetrakis(pentafluorophenyl)borate ethyl etherate (23 μmol, 20 eq.) dissolved in 1.6 ml of acetonitrile were added rapidly 1.9 mg of rhodamine B octadecyl ester perchlorate (2.4 μmol) in 0.4 ml acetonitrile. After evaporation of the solvent, the raw product was purified by thin layer chromatography (eluent: dichloromethane/methanol: 98/2). After re-dissolution, filtration and drying under vacuum, the product was obtained as a purple solid (2.3 mg, yield 70%). 1 H NMR (400 MHz, CD 3 OD): δ 8.31 (dd, J =7.6 Hz, J =2.1 Hz, 1H), 7.83 ( m , 2H), 7.43 (dd, J =7.3 Hz, J =1.2 Hz, 1H), 7.15 ( d , J =9.6 Hz, 2H), 7.04 (dd, J =9.6 Hz, J =2.3 Hz, 2H), 6.96 ( d , J =2.3 Hz, 2H), 3.94 ( t , J =6.3 Hz, 2H), 3.71 ( q , J =7.1 Hz, 8H), 1.32 ( t , J =7.0 Hz, 12H), 1.28–0.85 ( m , 35H); 13 C NMR (125 MHz, CD 3 OD): δ 166.9, 160.2, 159.3, 157.1, 149.4 ( d , J =241 Hz), 139.5 ( d , J =246 Hz), 137.5 ( d , J =246 Hz), 134.5, 133.9, 132.4, 132.3, 131.9, 131.5, 131.4, 125.6 ( m ), 115.5, 114.8, 97.2, 66.7, 46.8, 33.1, 30.8, 30.7, 30.5, 30.4, 30.3, 29.4, 26.9, 23.7, 14.4, 12.8; 11 B NMR (128 MHz, CD 3 OD): δ −16.7 ( m ); 19 F NMR (160 MHz, CD 3 OD): δ −134 ( m , 2F), −166 ( t , J =39.5 Hz, 1F), −169 ( m , 2F); HRMS ( m/z ): [M] + calcd. for C 46 H 67 N 2 O 3 , 695.5146; found, 695.5159; [M] − calcd. for C 24 BF 20 , 678.9779; found, 678.9769. Preparation of fluorescent NPs PLGA (lactide:glycolide, 1:1, mole:mole, M n 24 000) was dissolved at 2 mg ml −1 in acetonitrile containing different amounts of dye (from 0 to 5 wt% relative to the PLGA). These solutions were added quickly and under stirring (shaking) using a micropipette to a tenfold volume excess of 20 mM phosphate buffer at pH 7.4. The particle solution was then quickly diluted fivefold with the same buffer. Characterization of NPs DLS measurements were performed on a Zetasizer Nano series DTS 1060 (Malvern Instruments S.A.). Absorption and emission spectra were recorded on a Cary 400 Scan ultraviolet–visible spectrophotometer (Varian) and a FluoroMax-3 spectrofluorometer (Horiba Jobin Yvon) equipped with a thermostated cell compartment, respectively. For standard recording of fluorescence spectra, the excitation wavelength was set to 530 nm and emission was recorded from 540 to 700 nm. Steady-state anisotropy was measured on a SLM 8000 spectrofluorometer (Aminco) in a T-configuration. QYs were calculated using rhodamine B in methanol ( QY =0.70) with an absorbance of 0.01 at 530 nm as a reference [54] . Time-resolved fluorescence measurements were performed with the time-correlated, single-photon counting technique using the excitation pulses at 480 nm provided by a pulse-picked frequency-doubled Ti-sapphire laser (Tsunami, Spectra Physics) pumped by a Millenia X laser (Spectra Physics) [55] . The emission was collected through a polarizer set at the magic angle and an 8-nm band-pass monochromator (Jobin-Yvon H10) at 582 nm. The instrumental response function was recorded with a polished aluminium reflector, and its full-width at half-maximum was 40 ps. For time-resolved anisotropy measurements, the fluorescence decay curves were recorded at the vertical and horizontal positions of the excitation polarizer and with the emission polarizer set to the vertical position, and analysed by the following equation: where I v and I h are the intensities collected at vertical and horizontal excitation polarizations, respectively, and G is the geometry factor at the emission wavelength, determined in independent experiments. Time-resolved intensity data were treated with a non-linear least-square analysis using the maximum entropy method (MEM) [56] . In the case of 1 and 5 wt% F5-TPB NPs, meaningful fitting using this software could not be performed due to the very fast decay of the anisotropy. In these cases the residual anisotropy r ∞ was obtained as the mean value of the anisotropy between 1 and 4 ns. The error on the residual anisotropy was estimated as s.e.m. Fluorescence microscopy and AFM For single-particle fluorescence and AFM measurements, the NPs were immobilized on glass surfaces on which a polyethyleneimine layer was initially adsorbed. The solutions of NPs were diluted to a particle concentration of about 6 pM (30 pM for AFM without fluorescence microscopy) with buffer. Four hundred microlitres of these solutions per cm 2 were then brought in contact with the polyethyleneimine-covered glass for 15 min, followed by extensive rinsing with milliQ-water. The surfaces were left in milliQ-water during microscopy and AFM measurements. Quantum dots (QDot 605 streptavidine conjugate, Invitrogen) at 6 pM concentration were immobilized and imaged in the same way as PLGA NPs. Single-particle measurements were performed in the TIRF (Total Internal Reflection Fluorescence) mode on a home-made wide-field setup based on an Olympus IX-71 microscope with an oil immersion objective (numerical aperture=1.49, × 100). A DPPS (Cobolt) continuous wave laser emitting at 532 nm was used for excitation. The laser intensity was changed between 0.45 and 13.5 W cm −2 by using a polarizer and a half-wave plate (532 nm). The fluorescence signal was recorded with an EMCCD camera (ImagEM Hamamatsu). For the determination of the number of emitting fluorophores per NP, FluoSpheres red–orange (diameter 0.04 μm, carboxylate modified, Invitrogen) immobilized and imaged in the same way as the NPs were used as a reference. From the micrographs, the mean fluorescence intensity of the FluoSpheres I FS was determined. Their QY ( QY FS =0.57) and per-particle molar absorption coefficient ( ε FS =13,560,000 M −1 cm −1 at 532 nm) were determined in independent measurements. From this, the number N NP of emitting fluorophores in the NPs was obtained according to: where I NP is the emission intensity of the NPs, ε RhC18 is the molar absorption coefficient of R18 and QY RhC18 is its QY at the corresponding dye loading. On and off times of NPs were obtained through a threshold analysis. For this, the transients of at least 200 NPs per condition were analysed using R software (R Project for Statistical Computing, http://www.r-project.org/ ). NPs were considered to be in their off-state when the fluorescence was <20% of the maximum fluorescence of the NP. To obtain super-resolution images, raw images of single-particle signals were analysed with an ImageJ plugin developed by N. Stuurman (Localization Microscopy). In practice, for each individual frame, spatially separated point spread function signals emitted by single emitters were detected and fitted with a two-dimensional Gaussian distribution. Subsequently, super-resolution images were rendered by superimposing the position coordinates of the detected single emitters, represented with a two-dimensional Gaussian curve with the same intensity value, using an s.d. that had been previously determined by the localization accuracy of single emitters (typically 18 nm). The AFM/fluorescence microscopy consists a combination of an AFM composed of a SMENA Head driven by NTEGRA electronics (NT-MDT) implemented on a homemade wide-field fluorescence inverted microscope. The fluorescence microscope works in the TIRF mode and is based on an Olympus IX-71 inverted microscope with an oil immersion objective (numerical aperture=1.49, × 100). A DPPS (Cobolt) continuous wave laser emitting at 532 nm was used to excite the NPs with a power of 3 W cm − 2 . Fluorescence image acquisition was performed using an EMCCD camera IXON 897 (ANDOR Inc., UK). AFM images were made in the tapping mode, using an NSG03 (NT-MDT) cantilever tip with a typical spring constant of 1.1 N m −1 , in liquid environment. Cellular studies HeLa cells (ATCC CCL-2) were grown in DMEM (Gibco–Invitrogen), supplemented with 10% fetal bovine serum (Lonza) and 1% antibiotic solution (penicillin–streptomycin, Gibco–Invitrogen) at 37 °C in humidified atmosphere containing 5% CO 2 . Cells were seeded onto a chambered coverglass (IBiDi) at a density of 5 × 10 4 cells per well 24 h before the microscopy measurement. For imaging, the culture medium was removed and the attached cells were washed with Opti-MEM (Gibco–Invitrogen). Next, a freshly prepared solution of 1 wt% R18/F5-TPB NPs (at 0.15 nM of NPs) in Opti-MEM was added to the cells and incubated for different time periods. For co-localization with LysoTracker Green DND-26 (Life Technologies), cells were stained with 50 nM agent for 30 min at 37 °C before visualization on the microscope. Cell membrane staining with wheat-germ agglutinin-Alexa488 was done for 10 min at room temperature before the measurements. For cytotoxicity studies, HeLa cells were seeded in 96-well plates at a concentration of 10 4 cells per well in 100 μl of the DMEM growth medium and then incubated overnight at 37 °C in humidified atmosphere containing 5% CO 2 . Next, the PLGA NPs were added by substituting the culture medium for a similar one containing variable concentrations of NPs. After incubation for 24 or 78 h, the medium was removed and the adherent cell monolayers were washed with PBS. Next, the wells were filled with cell culture medium containing MTT (3-(4,5-dimethylthiazol-2-yl)-2,5-diphenyltetrazolium bromide), incubated for 4 h at 37 °C, and the formazan crystals formed were dissolved by adding 100 μl of a 10% SDS, 0.01 M hydrochloric acid solution. The absorbance was then measured at 570 nm with a microplate reader. Experiments were carried out in triplicate and expressed as the percentage of viable cells compared with the control group. How to cite this article: Reisch, A. et al. Collective fluorescence switching of counterion-assembled dyes in polymer nanoparticles. Nat. Commun. 5:4089 doi: 10.1038/ncomms5089 (2014).